Myeloid-derived interleukin-1β drives oncogenicKRAS-NF-κΒ addiction in malignant pleural effusion Malignant pleural effusion (MPE) is a frequent metastatic manifestation of human cancers. While we previously identified KRAS mutations as molecular culprits of MPE formation, the underlying mechanism remained unknown. Here, we determine that non-canonical IKKα-RelB pathway activation of KRAS -mutant tumor cells mediates MPE development and this is fueled by host-provided interleukin IL-1β. Indeed, IKKα is required for the MPE-competence of KRAS -mutant tumor cells by activating non-canonical NF-κB signaling. IL-1β fuels addiction of mutant KRAS to IKKα resulting in increased CXCL1 secretion that fosters MPE-associated inflammation. Importantly, IL-1β-mediated NF-κB induction in KRAS -mutant tumor cells, as well as their resulting MPE-competence, can only be blocked by co-inhibition of both KRAS and IKKα, a strategy that overcomes drug resistance to individual treatments. Hence we show that mutant KRAS facilitates IKKα-mediated responsiveness of tumor cells to host IL-1β, thereby establishing a host-to-tumor signaling circuit that culminates in inflammatory MPE development and drug resistance. Malignant pleural effusion (MPE) is one of the most challenging cancer-related disorders. It ranks among the top prevalent metastatic manifestations of tumors of the lungs, breast, pleura, gastrointestinal tract, urogenital tract, and hematopoietic tissues, killing an estimated two million patients worldwide every year and causing 126,825 admissions in U.S. hospitals in 2012 alone [1] , [2] . The presence of a MPE at diagnosis is an independent negative prognostic factor in patients with lung cancer and mesothelioma [3] , [4] . In addition, current therapies are non-etiologic and often ineffective, may cause further morbidity and mortality, and have not yielded significant improvements in survival [5] , [6] . To meet the pressing need for mechanistic insights into the pathobiology of MPE, we developed immunocompetent mouse models of the condition that unveiled inflammatory tumor-to-host signaling networks causing active plasma extravasation into the pleural space [7] . Nuclear factor (NF)-κB activity in tumor cells was pivotal for MPE formation in preclinical models, driving pro-inflammatory gene expression and promoting pleural tumor cell survival [8] , [9] , [10] . However, the mechanism of oncogenic NF-κB activation of MPE-competent pleural tumor cells remained unknown. In parallel, we recently pinned mutant KRAS as a molecular determinant of the propensity of pleural-metastasized tumor cells for MPE formation: mutant KRAS delivered its pro-MPE effects by directly promoting C-C chemokine motif ligand 2 (CCL2) secretion by pleural tumor cells, resulting in pleural accumulation of MPE-fostering myeloid cells [11] . However, a unifying mechanism linking KRAS mutations with oncogenic NF-κB activation and MPE competence of pleural tumor cells was missing. KRAS mutations have been previously linked to elevated or aberrant NF-κB activity via cell-autonomous and paracrine mechanisms. KRAS -mutant tumors, including lung and pancreatic adenocarcinomas, require active NF-κB signaling [12] , [13] , [14] and NF-κB inhibition blocks KRAS -induced tumor growth [14] , [15] , [16] . In turn, NF-κB activation of KRAS -mutant tumor cells has been associated with enhanced RAS signaling, drug resistance, and stemness [17] , [18] . Despite significant research efforts, the NF-κB-activating kinases (ΙκΒ kinases, IKK) and pathways (canonical, involving ΙκΒα, ΙΚΚβ, and Rel A/P50, versus non-canonical, comprising IκΒβ, ΙΚΚα, and Rel B/P52) that mediate this oncogenic addiction between mutant KRAS and NF-κB signaling are still elusive and diverse, and different studies indicate that IKKα, IKKβ, IKKγ, IKKε, and/or TANK-binding kinase 1 (TBK1) are key for this [17] , [18] , [19] , [20] , [21] , [22] , [23] , [24] . Here we use immunocompetent mouse models of MPE to show that mutant KRAS determines the responsiveness of pleural tumor cells to host-delivered interleukin (IL)-1β signals by directly regulating IL-1 receptor 1 (IL1R1) expression. IKKα is further shown to critically mediate IL-1β signaling in KRAS -mutant tumor cells, culminating in marked MPE-promoting effects delivered by C-X-C chemokine motif ligand 1 (CXCL1), and in oncogenic addiction with mutant KRAS evident as drug resistance. Importantly, simultaneous inhibition of IKKα and KRAS is effective in annihilating mutant KRAS -IKKα addiction in MPE. Non-canonical NF-κB signaling of KRAS -mutant cancer cells We first evaluated resting-state NF-κB activity of five mouse cancer cell lines with defined KRAS mutations and MPE capabilities in syngeneic C57BL/6 mice [11] : Lewis lung carcinoma (LLC; MPE-competent; Kras G12C ), MC38 colon adenocarcinoma (MPE-competent; Kras G13R ), AE17 malignant pleural mesothelioma (MPE-competent; Kras G12C ), B16F10 skin melanoma, and PANO2 pancreatic adenocarcinoma (both MPE-incompetent and Kras WT ) cells. Parallel transient transfection of these cell lines with reporter plasmids encoding Photinus Pyralis LUC under control of either a constitutive (p CAG.LUC ) or a NF-κB-dependent ( pNF-κB.GFP.LUC ; p NGL ) promoter [8] , [9] , [10] , [11] , [25] (Fig. 1a ) revealed that unstimulated NF-κB activity did not segregate by KRAS mutation status (Fig. 1b ). However, when PANO2 cells, a cell line with relatively low NF-κB activity, were transiently transfected with p Kras G12C , their NF-κΒ expression levels were elevated (Fig. 1c ). Moreover, KRAS mutant (MUT) cells displayed elevated DNA-binding activity of non-canonical NF-κB subunits P52 and Rel B by functional NF-κΒ enzyme-linked immunosorbent assay (ELISA) and enhanced nuclear immunofluorescent localization of Rel B compared with KRAS WT cells (Fig. 1d, e ). Immunoblotting of cytoplasmic and nuclear extracts revealed that KRAS MUT cells had increased levels of cytoplasmic Rel A and IκΒα and of nuclear Rel B, ΙκΒβ, and ΙΚΚα compared with Kras WT cells (Fig. 1f ). These results suggest that KRAS MUT cancer cells exhibit non-canonical endogenous NF-κB activity. Fig. 1 Kras -mutant tumor cells exhibit non-canonical endogenous NF-κΒ activity. Five different C57BL/6 mouse tumor cell lines with ( Kras MUT : LLC, MC38, AE17) or without ( Kras WT : B16F10, PANO2) Kras mutations were assessed for activation and inhibition of resting NF-κΒ activity in vitro. a Map of NF-κΒ reporter plasmid (NF-κΒ.GFP.Luc; p NGL ). Partial p NGL sequence at origin (1) showing κΒ-binding motifs (red) and GFP sequence (green). b Representative image and data summary ( n = 3) of area under curve of cumulative bioluminescence emitted by cells transiently transfected with reporter plasmids p CAG.LUC or p NGL . c Data summary ( n = 8) of bioluminescence emitted by PANO2 cells stably expressing p NGL reporter plasmid at 48 h after transient transfection with p C or p Kras G12C . d Data summary ( n = 5) of DNA NF-κB motif binding activity of nuclear extracts by NF-κB ELISA relative to nuclear extracts of Raji leukemia cells. e Immunofluorescent detection of Rel A and Rel B in cells grown on glass slides ( n = 3) showing increased nuclear localization of Rel B in Kras MUT cells and of Rel A in Kras WT cells (arrows). f Immunoblots of cytoplasmic and nuclear extracts for NF-κB pathway members and β-actin (representative of n = 3 independent experiments). Data presented as mean ± s.d. P , overall probability by one-way ( b ) and two-way ( d ) ANOVA or Student’s t -test ( c ). * P < 0.05 and *** P < 0.001 for the indicated comparisons by Bonferroni post-tests. g Data summary ( n = 3) of p NGL reporter activity after 4-h treatment and of cell proliferation by MTT assay after 72-h treatment in response to bortezomib, IMD-0354, or 17-DMAG. Data presented as mean ± s.d. from n = 3 replicates/data point. P , probability of no difference between cell lines by extra sum-of-squares F test. h , i Data summary of 50% inhibitory concentrations (IC 50 ) of NF-κΒ activity (by p NGL reporter activity) and cell proliferation (by MTT; g ). Data presented as mean ± s.d. from n = 3 independent experiments. P , probability of no difference by two-way ANOVA. ns and triple asterisks (***): P > 0.05 and P < 0.001, respectively, for the indicated comparisons by Bonferroni post-tests. nd not determined Full size image Resistance of KRAS -mutant cancer cells to IKKβ inhibition We next examined the effects of small molecule inhibitors of the proteasome (bortezomib [26] ), of IKKβ (IMD-0354 [27] ), or of heat shock protein 90 (HSP90) (17-dimethylaminoethylamino-17-demethoxygeldanamycin (17-DMAG) [28] ) that display significant inhibitory activity against IKKβ and/or IKKα (of note, a specific IKKα inhibitor does not exist) on NF-κB reporter activity and cellular proliferation of our murine cancer cell lines (Fig. 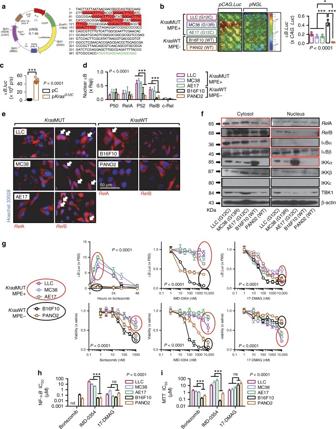Fig. 1 Kras-mutant tumor cells exhibit non-canonical endogenous NF-κΒ activity. Five differentC57BL/6mouse tumor cell lines with (KrasMUT: LLC, MC38, AE17) or without (KrasWT: B16F10, PANO2)Krasmutations were assessed for activation and inhibition of resting NF-κΒ activity in vitro.aMap of NF-κΒ reporter plasmid (NF-κΒ.GFP.Luc; pNGL). Partial pNGLsequence at origin (1) showing κΒ-binding motifs (red) and GFP sequence (green).bRepresentative image and data summary (n= 3) of area under curve of cumulative bioluminescence emitted by cells transiently transfected with reporter plasmids pCAG.LUCor pNGL.cData summary (n= 8) of bioluminescence emitted by PANO2 cells stably expressing pNGLreporter plasmid at 48 h after transient transfection with pCor pKrasG12C.dData summary (n= 5) of DNA NF-κB motif binding activity of nuclear extracts by NF-κB ELISA relative to nuclear extracts of Raji leukemia cells.eImmunofluorescent detection ofRelA andRelB in cells grown on glass slides (n= 3) showing increased nuclear localization ofRelB inKrasMUTcells and ofRelA inKrasWTcells (arrows).fImmunoblots of cytoplasmic and nuclear extracts for NF-κB pathway members and β-actin (representative ofn= 3 independent experiments). Data presented as mean ± s.d.P, overall probability by one-way (b) and two-way (d) ANOVA or Student’st-test (c). *P< 0.05 and ***P< 0.001 for the indicated comparisons by Bonferroni post-tests.gData summary (n= 3) of pNGLreporter activity after 4-h treatment and of cell proliferation by MTT assay after 72-h treatment in response to bortezomib, IMD-0354, or 17-DMAG. Data presented as mean ± s.d. fromn= 3 replicates/data point.P, probability of no difference between cell lines by extra sum-of-squaresFtest.h,iData summary of 50% inhibitory concentrations (IC50) of NF-κΒ activity (by pNGLreporter activity) and cell proliferation (by MTT;g). Data presented as mean ± s.d. fromn= 3 independent experiments.P, probability of no difference by two-way ANOVA. ns and triple asterisks (***):P> 0.05 andP< 0.001, respectively, for the indicated comparisons by Bonferroni post-tests. nd not determined 1g, h ; Supplementary Table 1 ). Bortezomib, an indirect inhibitor of IKKβ via cytoplasmic accumulation of non-degraded ΙκΒα [16] , [26] , attenuated endogenous NF-κB activity of Kras WT cells but paradoxically activated NF-κB in KRAS MUT cells, at the same time more effectively killing KRAS WT than KRAS MUT cells in vitro. Similarly, IKKβ-selective IMD-0354 [27] blocked NF-κB activity and cellular proliferation of unstimulated KRAS WT cells but not of KRAS MUT cells. Interestingly, the HSP90 and dual IKKα/IKKβ inhibitor 17-DMAG [29] was equally effective in limiting NF-κB activity and cellular proliferation of all cell lines irrespective of KRAS mutation status. These results suggest the existence of endogenous resistance of KRAS -mutant cells to IKKβ inhibition, which can be overcome by combined HSP90/IKKα/IKKβ inhibition. IL-1-inducible NF-κB activation of KRAS -mutant cancer cells We next studied NF-κB activation patterns of our murine cancer cells in response to exogenous stimuli. For this, cells were stably transfected with p NGL , were pretreated with saline or bortezomib (1 μM ~5–10-fold the 50% NF-κB inhibitory concentration obtained from Kras WT cells; Supplementary Table 1 ), were exposed to 60 different candidate NF-κB-pathway ligands at 1 nM concentration [30] , and were longitudinally monitored for NF-κB-dependent LUC activity by bioluminescence imaging of live cells in vitro (Fig. 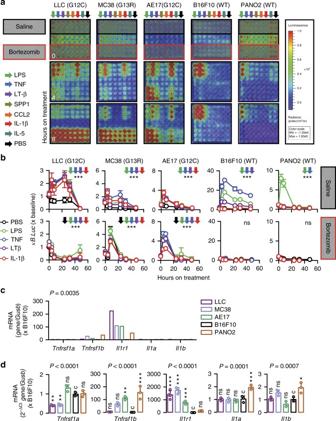Fig. 2 Kras-mutant tumor cells possess IL-1β-inducible NF-κΒ activity. Five differentC57BL/6mouse tumor cell lines with (LLC, MC38, AE17) or without (B16F10, PANO2)Krasmutations were assessed for inducible NF-κΒ activation in response to exogenous stimuli and for the expression of relevant receptors in vitro.a,bRepresentative bioluminescent images (a; shown aren= 3 replicates/data-point) and data summary (b; mean ± s.d. ofn= 3 independent experiments) of cells stably expressing pNGLand pretreated with saline or 1 μM bortezomib at different time points after addition of 1 nM of the indicated NF-κΒ ligands (arrows inaand legend inb). Note NF-κB inducibility by IL-1β and bortezomib exclusively inKrasMUTcells. ns and ***P> 0.05 andP< 0.001, respectively, for comparison between ligands indicated by colored arrows and PBS at 4 and 8 h on treatment by two-way ANOVA with Bonferroni post-tests.c,dTnfrsf1a,Tnfrsf1b,Il1r1,Il1a, andIl1bmRNA expression relative toGusbby microarray (c) and qPCR (d). Shown are mean (c) and mean ± s.d. (d) ofn= 5 independent technical replicates of one biologic sample.P, probability of no difference between cell lines by two-way (c) or one-way (d) ANOVA. ns, single, double, and triple asterisks (*, **, and ***):P> 0.05,P< 0.05,P< 0.01, andP< 0.001, respectively, for comparison with B16F10 cells (c) by Bonferroni post-tests 2a, b ; Supplementary Table 2 ). Incubation with lipopolysaccharide (LPS) and tumor necrosis factor (TNF) resulted in markedly increased NF-κB activity in all cells irrespective of KRAS status, while lymphotoxin β activated NF-κB in all but PANO2 cells, effects that peaked by 4–8 h of incubation and subsided by 16–24 h. Uniquely, IL-1α and IL-β induced NF-κB exclusively in KRAS MUT cells. In addition, bortezomib exaggerated endogenous and inducible NF-κB activation of KRAS MUT cells, in contrast to KRAS WT cells that displayed efficient NF-κΒ blockade by bortezomib. In line with the above, Il1r1 (encoding IL1R1, cognate to IL-1α/β) expression, but not Tnfrsf1a/Tnfrsf1b (encoding TNF receptors) or Il1a / Il1b expression (that was undetectable in all cell lines), was exclusively restricted to KRAS MUT MPE-proficient tumor cells (Fig. 2c, d ). We subsequently tested whether inducible NF-κB activation occurs in tumor cells entering the pleural space in vivo, simulating incipient pleural carcinomatosis [4] , [7] . For this, naive C57BL/6 mice were pulsed with a million intrapleural p NGL -expressing tumor cells and were serially imaged for NF-κB-dependent bioluminescence. Amazingly, KRAS MUT MPE-competent cells responded to the pleural environment with markedly escalated NF-κB activity within 4 h after injection, while KRAS WT MPE-incompetent cells showed diminishing NF-κB signals (Fig. 3a ). Interestingly, this in vivo NF-κB response of KRAS MUT cells was abolished in IL-1β-deficient ( Il1b−/− [31] ), but not in TNF-deficient ( Tnf−/− [32] ), mice (Fig. 3b ), indicating that KRAS MUT tumor cells selectively respond to IL-1β of the pleural environment by activating NF-κB. Fig. 2 Kras -mutant tumor cells possess IL-1β-inducible NF-κΒ activity. Five different C57BL/6 mouse tumor cell lines with (LLC, MC38, AE17) or without (B16F10, PANO2) Kras mutations were assessed for inducible NF-κΒ activation in response to exogenous stimuli and for the expression of relevant receptors in vitro. a , b Representative bioluminescent images ( a ; shown are n = 3 replicates/data-point) and data summary ( b ; mean ± s.d. of n = 3 independent experiments) of cells stably expressing p NGL and pretreated with saline or 1 μM bortezomib at different time points after addition of 1 nM of the indicated NF-κΒ ligands (arrows in a and legend in b ). Note NF-κB inducibility by IL-1β and bortezomib exclusively in Kras MUT cells. ns and *** P > 0.05 and P < 0.001, respectively, for comparison between ligands indicated by colored arrows and PBS at 4 and 8 h on treatment by two-way ANOVA with Bonferroni post-tests. c , d Tnfrsf1a , Tnfrsf1b , Il1r1 , Il1a , and Il1b mRNA expression relative to Gusb by microarray ( c ) and qPCR ( d ). Shown are mean ( c ) and mean ± s.d. ( d ) of n = 5 independent technical replicates of one biologic sample. P , probability of no difference between cell lines by two-way ( c ) or one-way ( d ) ANOVA. ns, single, double, and triple asterisks (*, **, and ***): P > 0.05, P < 0.05, P < 0.01, and P < 0.001, respectively, for comparison with B16F10 cells ( c ) by Bonferroni post-tests Full size image Fig. 3 Pleural IL-1β activates NF-κB in Kras -mutant tumor cells in vivo. Five different C57BL/6 mouse tumor cell lines with (LLC, MC38, AE17) or without (B16F10, PANO2) Kras mutations were assessed for inducible NF-κΒ activation in response to the pleural environment in vivo. a Representative bioluminescent images and data summary ( n = 6 mice/cell line) of C57BL/6 mice at 0 and 4 h after intrapleural injection of a million mouse tumor cells stably expressing pNGL . Note the marked induction of the bioluminescent signal emitted specifically by Kras MUT cells after 4 h. Note also the diminishing signal emitted by Kras WT cells. b Representative bioluminescent images and data summary (LLC: n = 6 mice/genotype; MC38: n = 7 mice/genotype) of C57BL/6 , Tnf−/− and Il1b−/− mice at 0 and 4 h after intrapleural injection of LLC or MC38 cells stably expressing pNGL . Note the marked induction of the bioluminescent signal in C57BL/6 mice, the borderline reduction of its inducibility in Tnf−/− mice, and the disappearance of signal inducibility in Ilb−/− mice. Data are presented as mean ± s.d. P , probability of no difference between cell lines or genotypes by one-way ANOVA. ns, single, double, and triple asterisks (*, **, and ***): P > 0.05, P < 0.05, P < 0.01, and P < 0.001, respectively, for the indicated comparisons by Bonferroni post-tests Full size image Mutant KRAS promotes non-canonical NF-κB signaling To define the role of mutant KRAS in the aberrant NF-κB activation patterns of KRAS MUT tumor cells, including non-canonical endogenous NF-κB activity, resistance to IKKβ inhibition, and IL-1β-inducibility, we undertook short hairpin RNA (shRNA)-mediated KRAS silencing (sh Kras ) and plasmid-mediated overexpression of a mutant dominant-negative form of ΙκΒα (p ΙκΒα DN; inhibits canonical NF-κΒ signaling) in KRAS MUT cell lines, as well as plasmid-mediated overexpression of mutant KRAS (p Kras G12C ) in KRAS WT cell lines [11] , [33] . Stable p ΙκΒ αDN expression in MC38 cells ( Kras G13R ) resulted in decreased Rel A and sustained Rel B nuclear-binding activity, while sh Kras did not affect Rel A but abolished Rel B nuclear-binding activity (Fig. 4a ). sh Kras also eliminated nuclear Rel B localization in these cells without affecting Rel A (Fig. 4b ) and abolished nuclear IKKα immunoreactivity of LLC ( Kras G12C ) and MC38 cells (Fig. 4c ). sh Kras expression reversed the endogenous resistance of MC38 cells to bortezomib and IMD-0354, rendering them as sensitive as KRAS WT cells (Fig. 4d, e ). In addition, sh Kras annihilated IL-1β-induced NF-κB transcriptional activity of p NGL -expressing LLC, MC38, and AE17 ( Kras G12C ) cells (Fig. 4f ), and p Kras G12C transmitted this phenotype to Kras WT PANO2 cells (Fig. 4g ). Importantly, sh Kras abrogated the in vivo NF-κB response of pleural-inoculated MC38 cells, which was reinstated in PANO2 cells by stable p Kras G12C expression (Fig. 4h, i ). In parallel, KRAS silencing in KRAS MUT cells significantly decreased, whereas p Kras G12C overexpression in KRAS WT cells significantly increased Il1r1 expression, as well as resting-state and IL-1β-inducible nuclear immunoreactivity for Rel B, IκΒβ, and ΙΚΚα (Fig. 4j–l ). Collectively, these data indicate that mutant KRAS induces non-canonical NF-κΒ signaling of cancer cells in unstimulated and IL-1β-stimulated conditions. Fig. 4 Mutant Kras drives basal and IL-1β-induced non-canonical NF-κB signaling and drug resistance. a Rel A and Rel B binding of nuclear extracts of MC38 cells stably expressing a control plasmid (p C ), a mutant dominant-negative form of ΙκΒα (p ΙκΒα DN), control shRNA (sh C ), or anti- Kras shRNA (sh Kras ) relative to Raji leukemia cells by NF-κB ELISA ( n = 3 experiments). b Immunofluorescent detection of Rel A and Rel B in MC38 cells showing increased nuclear Rel B (arrows) and its disappearance in cells expressing sh Kras . c IKKα immunoblots of cytoplasmic and nuclear extracts of LLC and MC38 cells expressing sh C or sh Kras . ( n = 3 experiments). d , e MTT data ( n = 3 replicates/data-point) and mean (95% CI) IC 50 values ( n = 3 experiments) of MC38 cells stably expressing sh C or sh Kras treated with bortezomib ( d ) or IMD-0354 ( e ) for 72 h. P , probability of no difference between cell lines by extra sum-of-squares F test. f , g Bioluminescent detection of NF-κΒ activity in Kras MUT ( f ) and Kras WT ( g ) cells stably expressing p NGL and the indicated vectors during 4-h incubation with PBS or 1 nM TNF or IL-1β ( n = 3 experiments). h , i Data summary ( h ; n = 6 mice/group) and images ( i ) of C57BL/6 mice at 0 and 4 h after intrapleural injection of MC38 or PANO2 cells stably expressing pNGL and the indicated vectors. j Il1r1 mRNA expression by qPCR of Kras MUT and Kras WT cells stably expressing the indicated vectors. k Immunoblots of protein extracts of MC38 and PANO2 cells stably expressing the indicated vectors for NF-κB members after 4-h incubation with PBS or 1 nM TNF or IL-1β ( n = 3 experiments). l The above extracts were subjected to EMSA. Super-shift EMSA was performed with the indicated antibodies. IgG antibody served as negative control. Data are presented as mean ± s.d. P , probability of no difference between cell lines by two-way ANOVA. Single, double, and triple asterisks (*, **, and ***): P < 0.05, P < 0.01, and P < 0.001, respectively, for comparison with p C or sh C ( a , f , h , j ) or with PBS ( g ) by Bonferroni post-tests Full size image IKKα in mutant KRAS- dependent MPE To define the NF-κB-activating kinase responsible for aberrant NF-κΒ signaling of KRAS MUT cancer cells, we stably expressed shRNAs specifically targeting IKKα, IKKβ, IKKε, and TBK1 transcripts ( Chuk , Ikbkb , Ikbke , and Tbk1 , respectively) in our p NGL -expressing cell lines and validated them (Fig. 5a ). In addition, we cloned these murine transcripts into an eukaryotic expression vector and generated stable transfectants of our cell lines. Interestingly, resting-state NF-κB transcriptional activity across KRAS MUT cells was markedly suppressed by sh Chuk but not by sh Ikbkb or sh Tbk1 , while sh Ikbke yielded minor NF-κΒ inhibition in MC38 and AE17 cells. On the contrary, endogenous NF-κΒ-mediated transcription of B16F10 cells was exclusively silenced by sh Ikbkb and, to a lesser extent, sh Ikbke , and of PANO2 cells by no shRNA (Fig. 5b ). In a reverse approach, overexpression of any kinase resulted in enhanced NF-κΒ activity in all KRAS MUT cells, of IKKβ only in B16F10 cells, and of no kinase in PANO2 cells (Fig. 5c ). In addition to intrinsic, IKKα also mediated IL-1β-inducible NF-κΒ activity of KRAS MUT tumor cells, since sh Chuk but not sh Ikbkb abolished IL-1β-induced NF-κB activity across KRAS MUT cell lines (Fig. 5d ). In line with the above, sh Chuk abolished the immunoreactivity of MC38 cell nuclear extracts for Rel B, ΙκΒβ, and IKKα, both at resting and IL-1β-stimulated states (Fig. 5e ). Taken together, these data suggest that KRAS -mutant cancer cells respond to pleural IL-1β via IKKα-mediated non-canonical NF-κB activation. Based on these results and our previous identification of the importance of KRAS mutations and NF-κΒ signaling in MPE development [8] , [9] , [10] , [11] , we hypothesized that IKKα is required for sustained NF-κΒ activation and MPE induction by pleural-homed KRAS MUT cancer cells. To test this, we injected IKK-silenced p NGL -expressing LLC cells ( Kras G12C ; MPE-competent) into the pleural space of C57BL/6 mice. Indeed, recipients of IKKα-silenced LLC cells displayed significant reductions in MPE incidence and volume, pleural inflammatory cell influx, and pleural tumor NF-κΒ activity and prolonged survival. IKKε silencing delivered more modest and equivocal beneficial effects, while IKKβ and TBK1 silencing had no impact (Fig. 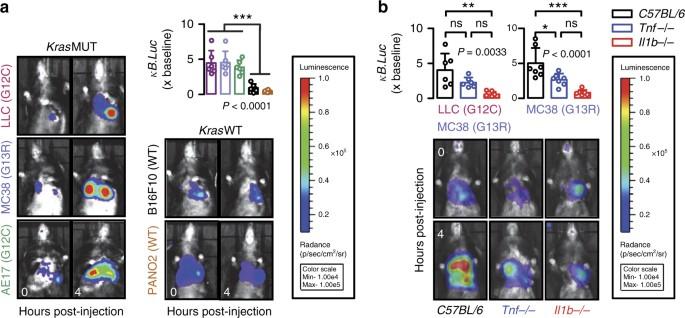Fig. 3 Pleural IL-1β activates NF-κB inKras-mutant tumor cells in vivo. Five differentC57BL/6mouse tumor cell lines with (LLC, MC38, AE17) or without (B16F10, PANO2)Krasmutations were assessed for inducible NF-κΒ activation in response to the pleural environment in vivo.aRepresentative bioluminescent images and data summary (n= 6 mice/cell line) ofC57BL/6mice at 0 and 4 h after intrapleural injection of a million mouse tumor cells stably expressingpNGL. Note the marked induction of the bioluminescent signal emitted specifically byKrasMUTcells after 4 h. Note also the diminishing signal emitted byKrasWTcells.bRepresentative bioluminescent images and data summary (LLC:n= 6 mice/genotype; MC38:n= 7 mice/genotype) ofC57BL/6,Tnf−/−andIl1b−/−mice at 0 and 4 h after intrapleural injection of LLC or MC38 cells stably expressingpNGL. Note the marked induction of the bioluminescent signal inC57BL/6mice, the borderline reduction of its inducibility inTnf−/−mice, and the disappearance of signal inducibility inIlb−/−mice. Data are presented as mean ± s.d.P, probability of no difference between cell lines or genotypes by one-way ANOVA. ns, single, double, and triple asterisks (*, **, and ***):P> 0.05,P< 0.05,P< 0.01, andP< 0.001, respectively, for the indicated comparisons by Bonferroni post-tests 6a–c ; Supplementary Table 3 ). These experiments were repeated with IKKα- and IKKβ-silenced MC38 cells ( Kras G13R ; MPE-competent) stably expressing p NGL , confirming that IKKα is cardinal for oncogenic NF-κΒ activation and MPE precipitation by pleural-metastatic KRAS MUT tumor cells (Fig. 6d–f ; Supplementary Table 3 ). However, standalone overexpression of IKKα or IKKβ did not confer MPE competence to KRAS WT PANO2 cells, as opposed to p Kras G12C (Fig. 6g–i ; Supplementary Table 3 ), in accord with our previous observations [11] . Collectively, these results suggest that mutant KRAS -potentiated IL-1β signaling results in KRAS MUT addiction to IKKα activity, which is required but not sufficient for oncogenic NF-κΒ activation and MPE formation. Fig. 5 IL-1β-induced NF-κB signaling of KRAS -mutant cells is IKKα dependent. Five different C57BL/6 mouse tumor cell lines with (LLC, MC38, AE17) or without (B16F10, PANO2) Kras mutations were stably transfected with p NGL NF-κΒ reporter and any of the following: control shRNA (sh C ) or shRNA targeting IKKα (sh Chuk ), ΙΚΚβ (sh Ikbkb ), ΙΚΚε (sh Ikbke ), or TBK1 (sh Tbk1 ) transcripts; control plasmid (p C ); or overexpression vectors encodong IKKα (p Chuk ), ΙΚΚβ (p Ikbkb ), ΙΚΚε (p Ikbke ), or TBK1 (p Tbk1 ) transcripts. a Immunoblot of cytoplasmic protein extracts from LLC cells stably expressing sh C , sh Chuk , or sh Ikbkb for IKKα and IKKβ relative to β-actin (representative of n = 3 independent experiments). b Bioluminescent quantification of NF-κΒ reporter activity of p NGL cell lines stably expressing sh C , sh Chuk , sh Ikbkb , sh Ikbke , and sh Tbk1 , ( n = 3 independent experiments). c Bioluminescent quantification of NF-κΒ reporter activity of p NGL cell lines stably expressing p C , p Chuk , p Ikbkb , p Ikbke , and p Tbk1 , ( n = 3 independent experiments). d Bioluminescent detection of NF-κΒ reporter activity in LLC, MC38, and AE17 cells ( Kras MUT ) stably expressing p NGL and sh C , sh Chuk , or sh Ikbkb ( n = 3 independent experiments) during 4-h incubation with 1 nM IL-1β. Note IL-1β-induced NF-κB activity of sh C and sh Ikbkb cells that is silenced in sh Chuk cells. e Immunoblots of cytoplasmic and nuclear protein extracts of MC38 cells stably expressing p NGL and sh C , sh Chuk , or sh Ikbkb after 4-h treatment with PBS, TNF, and IL-1β for various NF-κB pathway members and β-actin ( n = 3). Data are presented as mean ± s.d. of n = 3 independent experiments. P , probability of no difference between cell lines by two-way ANOVA. ns, single, double, and triple asterisks (*, **, and ***): P > 0.05, P < 0.05, P < 0.01, and P < 0.001, respectively, for comparison of color-coded sh or p with control sh or p within each cell line by Bonferroni post-tests Full size image Fig. 6 IKKα is required for mutant KRAS -induced malignant pleural effusion. a – c Malignant pleural disease induced by LLC cells ( Kras G12C ) stably expressing p NGL NF-κΒ reporter and control shRNA (sh C ) or shRNA targeting IKKα (sh Chuk ), ΙΚΚβ (sh Ikbkb ), ΙΚΚε (sh Ikbke ), or TBK1 (sh Tbk1 ) transcripts ( n is given in Table 3). Shown are Kaplan–Meier survival plot ( a ), data summaries of effusion volume and pleural fluid cells ( b ), and representative images of effusions (dashed lines) and pleural tumors (t) as well as bioluminescent images at day 13 after pleural injections of the indicated tumor cells ( c ). d – f Malignant pleural disease induced by MC38 cells ( Kras G13R ) stably expressing p NGL NF-κΒ reporter and sh C , sh Chuk , or sh Ikbkb ( n is given in Supplementary Table 3 ). Shown are immunoblots of cytoplasmic extracts ( d ), data summaries of effusion volume and pleural fluid cells ( e ), and representative images of effusions (dashed lines) and pleural tumors (t) as well as representative bioluminescent images at day 13 after pleural injections of the indicated tumor cells ( f ). g – i Malignant pleural disease induced by PANO2 cells ( Kras WT ) stably expressing p NGL NF-κΒ reporter and control plasmid (sh C ) or plasmid encoding IKKα (p Chuk ), ΙΚΚβ (p Ikbkb ), or mutant (p Kras G12C ) transcripts ( n is given in Supplementary Table 3 ). Shown are Kaplan–Meier survival plot ( g ), data summary of effusion volume ( h ), and representative images of effusions (dashed lines) and pleural tumors (t), hearts (h), and lungs (l), as well as representative bioluminescent images at day 14 after pleural injections of the indicated tumor cells ( i ). Data are presented as mean ± s.d. P , probability of no difference between cell lines by overall log-rank test ( a , g ) or one-way ANOVA ( b , e , h ). ns, single, double, and triple asterisks (*, **, and ***): P > 0.05, P < 0.05, P < 0.01, and P < 0.001, respectively, for the indicated comparisons with control cells by Bonferroni post-tests. Scale bars, 0.5 cm Full size image Myeloid IL-1β fosters mutant KRAS -IKKα addiction in MPE To study the importance of host-delivered IL-1β in the proposed KRAS MUT -IKKα addiction culminating in MPE, we delivered p NGL -expressing KRAS MUT LLC and MC38 cells into the pleural space of Il1b−/− , Tnf−/− , and WT C57BL/6 mice. Interestingly, Il1b−/− but not Tnf−/− mice displayed decreased MPE incidence, volume, inflammatory cell influx, and oncogenic NF-κB activation (Fig. 7a–d ; Supplementary Table 3 ). Host-provided IL-1β was of myeloid origin, since bone marrow (BM) transplants [34] , [35] from C57BL/6 and Tnf−/− , but not Il1b−/− donors, to lethally irradiated Il1b−/− recipients unable to foster MPE rendered LLC cells MPE proficient (Fig. 7e, f ; Supplementary Table 3 ). To define which myeloid cells provide the bulk of IL-1β to fuel tumor cell NF-κΒ activity, we isolated BM cells from C57BL/6 mice and drove them toward monocyte and neutrophil differentiation by macrophage colony-stimulating factor (M-CSF) and granulocyte-colony-stimulating factor (G-CSF culture, respectively. Both BM-derived monocytes and neutrophils secreted IL-1β upon 24-hour treatment with cell-free LLC supernatants as measured by ELISA, but monocytes secreted ~200 times higher cytokine levels than undifferentiated BM cells and neutrophils (Fig. 7g ). These data clearly show that the main source of IL-1β in the pleural space during MPE development likely are recruited myeloid monocyte cells. Fig. 7 Myeloid cell-derived IL-1β drives mutant KRAS -IKKα addiction in malignant pleural effusion. a Malignant pleural disease induced by LLC cells ( Kras G12C ) stably expressing p NGL NF-κΒ reporter plasmid in wild-type C57BL/6 mice (black) and TNF (blue) and IL-1β (red)-deficient mice ( Tnf−/− and Il1b −/−, respectively; both C57BL/6 background; n is given in Supplementary Table 3 ). Shown are data summaries of effusion volume, pleural fluid cells, and NF-κΒ-dependent thoracic bioluminescent signal. b – d Malignant pleural disease induced by MC38 cells ( Kras G13R ) stably expressing p NGL NF-κΒ reporter plasmid in wild-type C57BL/6 (black), Tnf−/− (blue), and Il1b−/− (red) mice (all C57BL/6 background; n is given in Supplementary Table 3 ). Shown are data summaries of effusion volume, pleural fluid cells, and NF-κΒ-dependent thoracic bioluminescent signal ( b ), representative images of effusions (dashed lines), pleural tumors (t), and lungs (l) ( c ), as well as representative bioluminescent images at day 13 after pleural injections of the indicated tumor cells ( d ). e , f Malignant pleural disease induced by LLC cells in Il1b−/− mice ( C57BL/6 background; n is given in Supplementary Table 3 ) that received total body irradiation (1100 Rad), same-day bone marrow transplants (10 million cells) from C57BL/6 (black), Tnf−/− (blue), or Il1b−/− (red) donors, and pleural tumor cells after 1 month. Shown are data summaries of effusion volume and pleural fluid cells ( e ) and representative images of effusions (dashed lines), pleural tumors (t), lungs (l), and hearts (h) ( f ). g IL-1β protein secretion by C57BL/6 mouse bone marrow-isolated myeloid cells 24 h after treatment with LLC supernatants; undifferentiated cells (day 0), neutrophils (day 2 after addition of 20 ng/ml G-CSF), and macrophages (day 6 after addition of 20 ng/ml M-CSF; n = 3 independent experiments). Data are presented as mean ± s.d. P , probability of no difference by one-way ANOVA. ns, single, double, and triple asterisks (*, **, and ***): P > 0.05, P < 0.05, P < 0.01, and P < 0.001, respectively, for the indicated comparisons by Bonferroni post-tests. Scale bars, 1 cm ( c , f ) and 100 μM ( g ) Full size image Mutant KRAS -IKKα addiction promotes MPE via CXCL1 secretion To identify the MPE effectors and transcriptional signatures of IL-1β/ KRAS /IKKα-addicted tumor cells, we subjected KRAS-silenced, IKKα-silenced, and IL-1β-challenged LLC and MC38 cells to microarray analyses, seeking for transcripts altered heterodirectionally by silencing/challenge. Thirty transcripts fulfilled these criteria in LLC (including Ppbp , encoding pro-platelet basic protein, PPBP, and Cxcl1 , encoding CXCL1) and 20 in MC38 (including Cxcl1 ) cells, with Cxcl1 being the only common gene of these two signatures (Fig. 8a, b ; Supplementary Tables 4 , 5 ). Cxcl1 microarray results were validated by quantitative PCR (qPCR) and ELISA (Fig. 8c–e ). Furthermore, chromatin immunoprecipitation (ChIP) was performed in LLC cells treated with phosphate-buffered saline (PBS) or IL-1β in order to specify whether and which NF-κB component directly binds to the promoter region of Cxcl1 . The data indicate that only Rel B and IKKα bind to the NF-κB element in the Cxcl1 promoter and that IL-1β significantly strengthens this binding (Fig. 8f ). These findings are consistent with the enhanced transcriptional induction of Cxcl1 . Moreover, Cxcl1 and Ppbp expression was pivotal for MPE induction by IL-1β/ KRAS /IKKα-addicted LLC cells, since these were MPE incompetent in both C-X-C chemokine motif receptor 1 (CXCR1) and CXCR2 gene-deficient mice [36] , [37] that lack the genes encoding CXCL1/PPBP-cognate CXCR1 and CXCR2 receptors [38] (Fig. 8g ; Supplementary Table 3 ). Notably, in MPEs from CXCR1 and CXCR2 gene-deficient mice the predominant cell population was monocytes, whereas in MPEs from CCR2 gene-deficient mice [11] the prevalent cell type was neutrophils. This result was not unexpected since the majority of myeloid cells recruited in the pleural space during MPE development in C57BL/6 mice consist of both neutrophils and monocytes (Fig. 8h ). Of note, the monocyte population is the most prevalent during MPE development. Fig. 8 CXCL1/PPBP are the downstream effectors of KRAS/IL-1β/IKKα signaling in malignant pleural effusion. a – c LLC and MC38 cells were stably transfected with sh C or sh Kras or shChuk or were stimulated with 1 nM IL-1β for 4 h, and total cellular RNA was examined by Affymetrix mouse gene ST2.0 microarrays. a Venn diagram of analytic strategy employed: transcripts altered >1.3-fold in one direction by sh Kras and sh Chuk and in the other by IL-1β were filtered for each cell line and are given in Supplementary Tables S1 – S2 . These gene sets, coined KRAS/IL-1β/IKKα signatures, were crossexamined and only Cxcl1 was common to both. b Unsupervised hierarchical clustering of LLC cell results by the 29-gene KRAS/IL-1β/IKKα signature accurately clustered three control samples together, sh Kras and sh Chuk samples together, and IL-1β-stimulated cells apart. c Cxcl1 mRNA normalized expression levels by microarray ( n = 2 independent experiments). d Cxcl1 mRNA expression by qPCR relative to Gusb ( n = 3 independent experiments). e CXCL1 protein secretion by LLC cells stably expressing sh C , sh Chuk , or sh Kras after 24 h of stimulation with PBS or 1 nM TNF or IL-1β ( n = 3 independent experiments). f Chromatin immunoprecipitation (ChIP) was performed in PBS- or IL-1β-treated LLC cells, followed by immunoprecipitation with the indicated antibodies. The immunoprecipitates were then detected by qPCR. Data are shown as fold enrichment of Cxcl1 or Gusb promoter in each antibody immunoprecipitate over control IgG immunoprecipitate. g Malignant pleural disease induced by LLC cells in C57BL/6 , Cxcr +/− , and Cxcr2 +/− mice ( n is given in Supplementary Table 3 ). Shown are data summaries of effusion volume and pleural fluid cells, as well as representative images of effusions (dashed lines), pleural tumors (t), lungs (l), and hearts (h). h Data summaries of C57BL/6 , Cxcr1 −/− , Cxcr2 +/− and Ccr2 −/− pleural neutrophils and monocytes, accompanied by microphotographs. Data are presented as mean ± s.d. P , probability of no difference by two-way ( c – e ) or one-way ( f – h ) ANOVA. ns, single, double, and triple asterisks (** and ***): P > 0.05, P < 0.05, P < 0.01, and P < 0.001, respectively, for comparison with PBS ( e ) or indicated ( g , h ) by Bonferroni post-tests. Scale bars 1 cm ( g ) and 200 μM ( h ) Full size image Combined targeting of KRAS /IKKα is effective against MPE To explore the therapeutic implications of the proposed mechanism, we examined potential synergy of the KRAS inhibitor deltarasin [39] with the IKKβ-specific inhibitor IMD-0354 or the HSP90/IKKα/IKKβ inhibitor 17-DMAG using TNF- or IL-1β-stimulated LLC murine and A549 human lung adenocarcinoma cells expressing p NGL (Fig. 9a, b ). Interestingly, all inhibitors alone or in combination failed to block TNF-inducible NF-κΒ activation in both cell lines. In addition, all standalone drugs failed to inhibit IL-1β-inducible NF-κΒ activation in both cell lines, except from partial effects observed in A549 cells by 17-DMAG. However, deltarasin/17-DMAG but not deltrarasin/IMD-0354 combination treatment completely abolished IL-1β-induced NF-κB activation in both cell types to unstimulated levels (Fig. 9a, b ), indicating that drugging the KRAS /IKKα axis can halt IL-1β responsiveness. To determine the potential efficacy of this approach against MPE, standalone or combined deltarasin, and 17-DMAG treatments (both 15 mg/Kg) were delivered to mice with established pleural tumors. For this, C57BL/6 mice received pleural LLC cells and treatments commenced after 5 days to allow initial pleural tumor implantation [11] . At day 13 post-tumor cells, standalone deltarasin and 17-DMAG-treated mice had significantly decreased MPE volume compared with saline-treated controls (40% reductions for both groups; P < 0.05; one-way analysis of variance (ANOVA) with Bonferroni post-tests). However, combination-treated mice were markedly protected from MPE development (57% incidence) and progression (65% volume reduction; P < 0.001; one-way ANOVA with Bonferroni post-tests) (Fig. 9c ; Supplementary Table 3 ). Hence combined targeting of mutant KRAS and IKKα is effective in halting oncogenic NF-κΒ activation and MPE in mice. Fig. 9 Combined targeting of mutant KRAS and IKKα abolishes IL-1β-induced NF-κΒ activation and malignant pleural effusion development. a , b Bioluminescent detection of NF-κΒ reporter activity in LLC ( a ; C57BL/6 Lewis lung carcinoma, Kras G12C ) and A549 ( b ; human lung adenocarcinoma, Kras G12S ) cells stably expressing p NGL under PBS or 1 nM TNF- or IL-1β-stimulated conditions (4 h), with or without pretreatment with 1 μM deltarasin, IMD-0354, or 17-DMAG alone or in combination ( n = 3 independent experiments). Note four-fold induction of NF-κΒ reporter activity by both TNF and IL-1β. Note also inability of any treatment to block TNF-induced NF-κΒ activation and of any standalone treatment except 17-DMAG to inhibit IL-1β-induced NF-κΒ activation. Finally, note complete abrogation of IL-1β-induced NF-κΒ activation in both cell lines by deltarasin/17-DMAG combination. Data are presented as mean ± s.d. P , probability of no difference by one-way ANOVA (PBS group excluded). Double and triple asterisks (** and ***): P < 0.01 and P < 0.001, respectively, for comparison with PBS by Student’s t -tests. Single and double section symbols (§ and §§): P < 0.05 and P < 0.01, respectively, for comparison with TNF or IL-1β by Bonferroni post-tests. c Malignant pleural disease induced by LLC cells in wild-type C57BL/6 mice treated with deltarasin and/or 17-DMAG. Mice received pleural LLC cells, were allowed 5 days for pleural tumor development, and were randomized to daily intraperitoneal treatments with saline (100 μL), deltarasin, 17-DMAG, or both (both at 15 mg/Kg in 100 μL saline; n is given in Supplementary Table 3 ). Shown are data summaries of effusion volume and pleural fluid cells and Kaplan–Meier survival plot, as well as representative images of effusions (dashed lines), pleural tumors (t), lungs (l), and hearts (h). Data are presented as mean ± s.d. P , probability of no difference by one-way ANOVA or log-rank test. ns, single, double, and triple (*, **, and ***): P > 0.05, P < 0.05, P < 0.01, and P < 0.001, respectively, for the indicated comparisons by Bonferroni post-tests. Scale bars, 1 cm Full size image IL-1β-inducible NF-κΒ activity in human KRAS -mutant cells To assess whether our findings are relevant to human cancer, we screened nine human cancer cell lines of known KRAS mutation status [40] for Rel -binding activity of nuclear extracts. In accord with murine data, KRAS MUT cells displayed enhanced nuclear Rel B compared with Rel A binding (Fig. 10a ). In addition, A549 ( KRAS G12S ) and NCI-H23 ( KRAS G12C ) cells displayed IL-1β-induced NF-κΒ activation, as opposed to HT-29 and SKMEL2 cells (both KRAS WT ). Importantly, stable p Kras G12C expression in SKMEL2 cells rendered them responsive to IL-1β (Fig. 10b, c ). Fig. 10 Non-canonical endogenous and IL-1β-inducible NF-κB activation of KRAS -mutant human tumor cells. Different human cancer cell lines with ( KRAS MUT : A549, KRAS G12S ; CCRF-CEM, KRAS G12D ; NCI-H23, KRAS G12C ) or without ( KRAS WT ; HT29, SKMEL2, MCF7, IGROV1, PC3, and M14K) KRAS mutations were assessed for NF-κΒ activation at resting and stimulated conditions in vitro. a Data summary ( n = 5 independent experiments) of DNA NF-κB motif-binding activity of nuclear extracts by NF-κB ELISA relative to nuclear extracts of Raji leukemia cells. Note increased nuclear Rel B and P52 binding activity of KRAS MUT compared with KRAS WT cells. b , c Bioluminescent detection of NF-κΒ reporter activity in A549, NCI-H23, HT29, and SKMEL2 cells stably expressing p NGL , as well as in SKMEL2 cells stably expressing p NGL and p Kras G12C ( b ; data summary of n = 5 independent experiments; c : representative bioluminescent images) during 4-h incubation with PBS or 1 nM TNF, IL-1β, or lymphotoxin (LT)-β. Note IL-1β-induced NF-κB activity of KRAS MUT but not of KRAS WT cells. Note also instalment of IL-1β-induced NF-κB activation in SKMEL2 cells by p Kras G12C (SKMEL2 cells expressing p C behaved exactly as parental cells). Data are presented as mean ± s.d. P , probability of no difference by two-way ANOVA. Triple astrisks (***): P < 0.001 for comparison with Rel A ( a ) or PBS ( b ) by Bonferroni post-tests Full size image In summary, KRAS mutations alter NF-κΒ signaling in tumor cells. KRAS WT cells preferentially utilize intrinsically or exogenously (i.e., by LPS, TNF) stimulated IKKβ-mediated NF-κΒ signaling, display sensitivity to IKKβ inhibition, poor CXCR1/2 ligand secretion, and MPE incompetence. KRAS MUT cells predominantly use IKKα-mediated non-canonical NF-κΒ signaling at resting state and in response to myeloid IL-1β, display enhanced CXCR1/2 ligand secretion and MPE proficiency, and are addicted to sustained IKKα activity evident as resistance to IKKβ inhibitors. We provide a novel paradigm of how an oncogene can co-opt the host environment to foster addiction with a perturbed signaling pathway. KRAS -mutant cancer cells are shown to respond to host provided IL-1β in the pleural space by increasing non-canonical IKKα-RelB pathway activity. The co-existence of mutant KRAS and elevated IKKα-mediated non-canonical NF-κB signaling in the cancer cell, relentlessly driven by host IL-1β, leads to two important consequences. First, to enhanced transcription of CXCL1/PPBP chemokines, recruitment of CXCR1+ and CXCR2+ myeloid cells, and frank escalation of inflammatory MPE development. Second, to oncogenic addiction between mutant KRAS and IKKα that culminates in drug resistance. Using immunocompetent mouse models of MPE, we show how IL-1β, mutant KRAS , and IKKα interplay to mediate non-canonical NF-κB activation, resistance to proteasome and IKKβ inhibitors, CXCL1/PPBP secretion, and MPE. Finally, we show that this partnership can be annihilated by combined inhibition of KRAS together with IKKα but not alone. Although cell-autonomous pro-tumorigenic functions of mutant KRAS are well charted [41] , [42] , [43] , mechanisms utilized by the oncogene to co-opt host cells from the tumor microenvironment in order to favor tumor progression have only recently begun to be elucidated. In this regard, mutant KRAS was first shown to promote chemokine secretion by tumor-initiated cells, thereby promoting tumor-associated inflammation [44] , [45] . Along similar lines, we recently showed that the oncogene is responsible for CCL2 secretion by pleural metastatic cancer cells, fostering inflammatory MPE formation [11] . Our present findings expand the paradigm of how mutant KRAS impacts tumor–host interactions: it renders tumor cells capable of sensing inflammatory IL-1β signals originating from the CCL2-recruited monocytes. The increased Il1r1 expression in these cells could be a result of IL-1β -induced phosphorylation by nuclear IKKa of Ser10 in histone H3 that could be especially important for subsequent modifications in a variety of genes, including Il1r1 . Moreover, integrated by IKKα-mediated non-canonical NF-κΒ activity, IL-1β signaling culminates in enhanced CXCL1/PPBP expression and secretion that function to escalate tumor-associated inflammation required for MPE. Hence, in addition to directly promoting chemokine expression, mutant KRAS is shown here to amplify host-originated inflammatory signals in order to escalate MPE-promoting inflammation. Mutant KRAS is known to enhance oncogenic NF-κB activity; however, it was mainly linked to IKKβ, ΙΚΚε, and TBK1 function [12] , [14] , [17] , [18] , [21] , [23] , [24] , [43] , and only two studies identified IKKα as an accessory to IKKβ in KRAS -mutant lung adenocarcinoma [22] and epidermal growth factor receptor-driven head and neck cancers [19] . Here we show for the first time that KRAS- mutant cancer cells display altered NF-κΒ utilization in resting and stimulated states, a phenomenon previously identified in pancreatic β cells [46] . Indeed, KRAS -mutant cancer cells displayed non-canonical endogenous NF-κΒ activity evident by enhanced nuclear localization and/or DNA-binding activity of Rel B, ΙκΒβ, and ΙΚΚα, which was further inducible by exogenous IL-1β. Importantly, non-canonical NF-κΒ utilization by KRAS -mutant cancer cells was IKΚα driven, involved RelB activation, and was required for MPE. Nuclear IKΚα functions have been identified previously, including histone 3 modifications augmenting TNF and receptor activator of NF-κB ligand-induced gene expression and repression of maspin, a metastasis gate-keeper [47] , [48] , [49] . Our work links IKKα function with IL-1β-induced RelB activation and CXCL1/PPBP transcription. Moreover, we provide novel evidence that mutant KRAS is indirectly responsible for non-canonical NF-κB activation, which is IKKa and RelB based, via sensitization of cancer cells to host IL-1β. Finally, IKKα is found to be responsible for MPE, an important metastatic manifestation of various cancers. The findings concur with previous reports of a combined requirement for IKKα and IKKβ for oncogenic NF-κB activation [19] , [22] , as well as with human observations of predominant non-canonical NF-κB activity of tumors with high incidence of KRAS mutations, such as lung adenocarcinoma [50] . However, we demonstrate an isolated requirement for IKKα in KRAS -driven MPE, an important cancer phenotype. In recent years, inflammation was established as a conditional tumor promoter [51] . IL-1α/β are important components of the tumor microenvironment that stimulate tumor invasiveness and angiogenesis [52] . Myeloid-derived IL-1β is implicated in the resistance to NF-κΒ inhibitors and IL-1β antagonism yielded beneficial effects in a mouse model of KRAS -mutant pancreatic cancer [53] , [54] . We found previously that IL-1α/β are present in human and experimental MPE and that MPE-competent adenocarcinomas trigger myeloid cells to secrete IL-1β [35] . Here the mechanism of pleural IL-1β function in MPE promotion is elucidated: CCL2-attracted monocyte-released IL-1β fosters NF-κΒ activation of MPE-prone KRAS -mutant carcinomas by potentiating non-canonical NF-κB signaling via IKKα. Undoubtedly, IL-1β is not the sole NF-κΒ ligand expressed in the malignancy-affected pleural space: TNF, a known stimulator of canonical NF-κB signaling, is present in MPE and promotes disease progression [9] . However, TNF likely originates from tumor cells in MPE [9] and non-specifically triggers NF-κB activation in any tumor type irrespective of its KRAS status and MPE competence, suggesting it functions as an autocrine growth factor across tumor types. On the contrary, IL-1α/β selectively fostered MPE competence of KRAS -mutant carcinomas, in agreement with previous reports of IL-1β-induced NF-κB activation independent from IKKβ [55] . Our findings explain how the tumor microenvironment fuels tumor NF-κΒ activity [56] and link the pro-tumorigenic functions of IL-1β with KRAS mutations, setting a rationale for genotype-stratified future investigations on IL-1β functions and therapies in cancer. Unbiased analyses identified cancer-elaborated CXCL1/PPBP, potent myeloid cell chemoattractants that drive inflammation and metastasis via CXCR1/CXCR2 on host cells [57] , [58] , as the transcriptional targets of IL-1β-fostered KRAS -IKKα addiction. Indeed, Cxcl1 expression was downregulated by Kras or Chuk silencing and IL-1β induced Cxcl1 expression by two different cancer cell lines and Ppbp by LLC cells (MC38 cells do not express Ppbp [25] ). Our experiments using CXCR1- and CXCR2-deficient mice support that pleural tumor cell-secreted CXCL1/PPBP is cardinal for MPE and are in line with a previous study demonstrating increased production of CXCL1 by tumor cells during human MPE development that mobilizes regulatory T cells [59] . In addition to the mechanistic insights into host environment-fostered co-option of IKKα activity by mutant KRAS , our data bear therapeutic implications for KRAS inhibitors [39] . KRAS is notoriously undruggable, and proteasome and IKKβ inhibitors have yielded suboptimal results in mice and men with cancer. Focusing on lung cancer, a tumor with high KRAS mutation frequency [60] , bortezomib has shown poor efficacy in clinical trials [61] . In animal models of lung cancer, bortezomib and IKKβ inhibitors caused resistance or paradoxical tumor promotion via development of secondary mutations, NF-κB inhibition in myeloid cells, or enhanced IL-1β secretion by tumor-associated neutrophils through an unknown mechanism [15] , [16] , [53] . We show how KRAS -mutant cancer cells utilize myeloid-IL-1β in order to activate IKKα and alternative NF-κB signaling and to by-pass IKKβ canonical NF-κB dependence. We provide proof-of-concept data that KRAS -mutant cancer cells can be targeted by combined inhibition of KRAS and HSP90/IKKα/IKKβ signaling, a strategy that blocks IL-1β-inducible oncogenic NF-κB activation and in vivo MPE development, a cancer phenotype that requires mutant KRAS -potentiated, IL-1β-induced IKKα activity. These results challenge the prevailing focus on IKKβ for the development of anti-tumor drugs and establish IL-1β and IKKα as important targets in KRAS -mutant tumors. In conclusion, we show that KRAS -mutant cancer cells use host IL-1β to sustain IKKα-mediated non-canonical NF-κB activity responsible for MPE development and primary drug resistance. We identify CXCL1/PPBP as effectors of MPE downstream of KRAS /IKKα addiction. Finally, we provide proof-of-concept data suggesting that KRAS /IKKα addiction may occur in human cancers and may be targeted by combined KRAS /IKKα inhibition. Study approval All mouse experiments were prospectively approved by the Veterinary Administration of Western Greece (approval # 276134/14873/2) and were conducted according to Directive 2010/63/EU ( http://eur-lex.europa.eu/legal-content/EN/TXT/?uri=celex%3A32010L0063 ). Reagents D-Luciferin was from Gold Biotechnology (St. Louis, MO); lentiviral shRNA and puromycin from Santa Cruz (Dallas, TX); 3-(4,5-dimethylthiazol-2-yl)-2,5-diphenyltetrazolium bromide (MTT) assay and Hoechst 33528 from Sigma-Aldrich (St. Louis, MO); mouse gene ST2.0 microarrays and relevant reagents from Affymetrix (Santa Clara, CA); recombinant cytokines and growth factors from Immunotools (Friesoythe, Germany); NF-κB-binding ELISA from Active Motif (La Hulpe, Belgium); bortezomib, IMD-0354, 17-DMAG, and deltarasin from Selleckchem (Houston, TX); G418 from Applichem (Darmstadt, Germany); IL-1β and CXCL1 ELISA from Peprotech (London, UK); and primers from VBC Biotech (Vienna, Austria). Primers, antibodies, and lentiviral shRNA pools are listed in Supplementary Tables 6 – 8 . Cells LLC, B16F10, PANO2, and A549 cells were from the National Cancer Institute Tumor Repository (Frederick, MD); MC38 cells were a gift from Dr. Barbara Fingleton (Vanderbilt University, Nashville, TN) [34] , [35] , and AE17 cells from Dr. YC Gary Lee (University of Western Australia, Perth, Australia) [11] , [25] . All cell lines were cultured at 37 °C in 5% CO 2 –95% air using Dulbecco’s modified Eagle’s medium (DMEM) containing 10% fetal bovine serum, 2 mM L-glutamine, 1 mM pyruvate, 100 U/mL penicillin, and 100 mg/mL streptomycin. Cell lines were tested annually for identity by short tandem repeats and for Mycoplasma Spp. by PCR. For in vivo injections, cells were harvested using trypsin, incubated with Trypan blue, counted in a hemocytometer, and 95% viable cells were injected intrapleurally [8] , [11] , [34] , [35] . Mouse models and drug treatments C57BL/6 (#000664), B6.129P2- Cxcr1 tm1Dgen /J ( Cxcr1 −/− ; #005820 [36] ), B6.129 S2(C)-C xcr2 tm1Mwm /J ( Cxcr2 +/− ; #006848 [37] ), B6;129S- Tnf tm1Gkl /J ( Tnf−/− ; #003008 [32] ) (Jackson Laboratory, Bar Harbor, ME), and Il1b tm1Yiw ( Il1b −/− ; MGI #2157396 [31] ) mice were bred at the Center for Animal Models of Disease of the University of Patras. Male and female experimental mice and littermate controls were sex, weight (20–25 g), and age (6–12 weeks) matched. For MPE induction, mice received 150,000 cancer cells in 100 μL PBS intrapleurally. Mice were observed continuously till recovery and daily thereafter and were sacrificed when moribund (13–14 days post-tumor cells) for survival and pleural fluid analyses. Mice with pleural fluid volume ≥100 μL were judged to have a MPE and were subjected to pleural fluid aspiration, whereas animals with pleural fluid volume <100 μL were judged not to have a MPE and were subjected to pleural lavage. Injection, harvest, and sample handling are described elsewhere [8] , [9] , [10] , [11] , [34] , [35] . Drug treatments were initiated 5 days post-tumor cells and consisted of daily intraperitoneal injections of 100 μL PBS containing no drug, deltarasin [39] , 17-DMAG [28] , or both at 15 mg/kg. Constructs p NGL , p ΙκΒα DN, and p CAG.LUC (#74409) have been described elsewhere [8] , [25] , [33] . Lentiviral shRNA pools (Santa Cruz) are described in Supplementary Table 8 . A p MIGR1 -based (#27490) bicistronic retroviral expression vector was generated by replacing eGFP sequences with puromycin resistance gene (#58250). 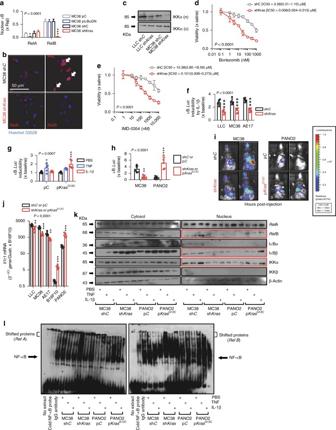Fig. 4 MutantKrasdrives basal and IL-1β-induced non-canonical NF-κB signaling and drug resistance.aRelA andRelB binding of nuclear extracts of MC38 cells stably expressing a control plasmid (pC), a mutant dominant-negative form of ΙκΒα (pΙκΒαDN), control shRNA (shC), or anti-KrasshRNA (shKras) relative to Raji leukemia cells by NF-κB ELISA (n= 3 experiments).bImmunofluorescent detection ofRelA andRelB in MC38 cells showing increased nuclearRelB (arrows) and its disappearance in cells expressing shKras.cIKKα immunoblots of cytoplasmic and nuclear extracts of LLC and MC38 cells expressing shCor shKras. (n= 3 experiments).d,eMTT data (n= 3 replicates/data-point) and mean (95% CI) IC50values (n= 3 experiments) of MC38 cells stably expressing shCor shKrastreated with bortezomib (d) or IMD-0354 (e) for 72 h.P, probability of no difference between cell lines by extra sum-of-squaresFtest.f,gBioluminescent detection of NF-κΒ activity inKrasMUT(f) andKrasWT(g) cells stably expressing pNGLand the indicated vectors during 4-h incubation with PBS or 1 nM TNF or IL-1β (n= 3 experiments).h,iData summary (h;n= 6 mice/group) and images (i) ofC57BL/6mice at 0 and 4 h after intrapleural injection of MC38 or PANO2 cells stably expressingpNGLand the indicated vectors.jIl1r1mRNA expression by qPCR ofKrasMUTandKrasWTcells stably expressing the indicated vectors.kImmunoblots of protein extracts of MC38 and PANO2 cells stably expressing the indicated vectors for NF-κB members after 4-h incubation with PBS or 1 nM TNF or IL-1β (n= 3 experiments).lThe above extracts were subjected to EMSA. Super-shift EMSA was performed with the indicated antibodies. IgG antibody served as negative control. Data are presented as mean ± s.d.P, probability of no difference between cell lines by two-way ANOVA. Single, double, and triple asterisks (*, **, and ***):P< 0.05,P< 0.01, andP< 0.001, respectively, for comparison with pCor shC(a,f,h,j) or with PBS (g) by Bonferroni post-tests 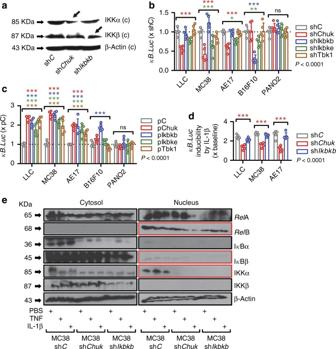Fig. 5 IL-1β-induced NF-κB signaling ofKRAS-mutant cells is IKKα dependent. Five differentC57BL/6mouse tumor cell lines with (LLC, MC38, AE17) or without (B16F10, PANO2)Krasmutations were stably transfected with pNGLNF-κΒ reporter and any of the following: control shRNA (shC) or shRNA targeting IKKα (shChuk), ΙΚΚβ (shIkbkb), ΙΚΚε (shIkbke), or TBK1 (shTbk1) transcripts; control plasmid (pC); or overexpression vectors encodong IKKα (pChuk), ΙΚΚβ (pIkbkb), ΙΚΚε (pIkbke), or TBK1 (pTbk1) transcripts.aImmunoblot of cytoplasmic protein extracts from LLC cells stably expressing shC, shChuk, or shIkbkbfor IKKα and IKKβ relative to β-actin (representative ofn= 3 independent experiments).bBioluminescent quantification of NF-κΒ reporter activity of pNGLcell lines stably expressing shC, shChuk, shIkbkb, shIkbke, and shTbk1, (n= 3 independent experiments).cBioluminescent quantification of NF-κΒ reporter activity of pNGLcell lines stably expressing pC, pChuk, pIkbkb, pIkbke, and pTbk1, (n= 3 independent experiments).dBioluminescent detection of NF-κΒ reporter activity in LLC, MC38, and AE17 cells (KrasMUT) stably expressing pNGLand shC, shChuk, or shIkbkb(n= 3 independent experiments) during 4-h incubation with 1 nM IL-1β. Note IL-1β-induced NF-κB activity of shCand shIkbkbcells that is silenced in shChukcells.eImmunoblots of cytoplasmic and nuclear protein extracts of MC38 cells stably expressing pNGLand shC, shChuk, or shIkbkbafter 4-h treatment with PBS, TNF, and IL-1β for various NF-κB pathway members and β-actin (n= 3). Data are presented as mean ± s.d. ofn= 3 independent experiments.P, probability of no difference between cell lines by two-way ANOVA. ns, single, double, and triple asterisks (*, **, and ***):P> 0.05,P< 0.05,P< 0.01, andP< 0.001, respectively, for comparison of color-coded sh or p with control sh or p within each cell line by Bonferroni post-tests 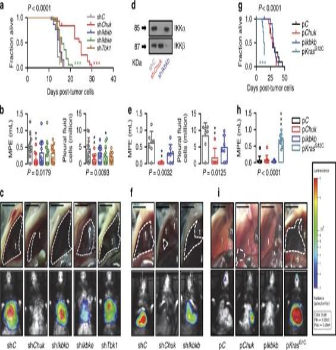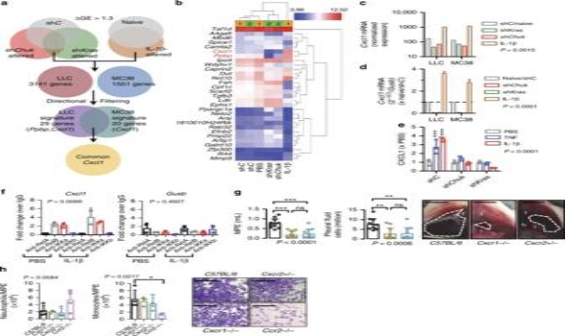Fig. 8 CXCL1/PPBP are the downstream effectors of KRAS/IL-1β/IKKα signaling in malignant pleural effusion.a–cLLC and MC38 cells were stably transfected with shCor shKrasor shChuk or were stimulated with 1 nM IL-1β for 4 h, and total cellular RNA was examined by Affymetrix mouse gene ST2.0 microarrays.aVenn diagram of analytic strategy employed: transcripts altered >1.3-fold in one direction by shKrasand shChukand in the other by IL-1β were filtered for each cell line and are given in Supplementary TablesS1–S2. These gene sets, coined KRAS/IL-1β/IKKα signatures, were crossexamined and onlyCxcl1was common to both.bUnsupervised hierarchical clustering of LLC cell results by the 29-gene KRAS/IL-1β/IKKα signature accurately clustered three control samples together, shKrasand shChuksamples together, and IL-1β-stimulated cells apart.cCxcl1mRNA normalized expression levels by microarray (n= 2 independent experiments).dCxcl1mRNA expression by qPCR relative toGusb(n= 3 independent experiments).eCXCL1 protein secretion by LLC cells stably expressing shC, shChuk, or shKrasafter 24 h of stimulation with PBS or 1 nM TNF or IL-1β (n= 3 independent experiments).fChromatin immunoprecipitation (ChIP) was performed in PBS- or IL-1β-treated LLC cells, followed by immunoprecipitation with the indicated antibodies. The immunoprecipitates were then detected by qPCR. Data are shown as fold enrichment ofCxcl1orGusbpromoter in each antibody immunoprecipitate over control IgG immunoprecipitate.gMalignant pleural disease induced by LLC cells inC57BL/6,Cxcr+/−, andCxcr2+/−mice (nis given in Supplementary Table3). Shown are data summaries of effusion volume and pleural fluid cells, as well as representative images of effusions (dashed lines), pleural tumors (t), lungs (l), and hearts (h).hData summaries ofC57BL/6,Cxcr1−/−,Cxcr2+/−andCcr2−/−pleural neutrophils and monocytes, accompanied by microphotographs. Data are presented as mean ± s.d.P, probability of no difference by two-way (c–e) or one-way (f–h) ANOVA. ns, single, double, and triple asterisks (** and ***):P> 0.05,P< 0.05,P< 0.01, andP< 0.001, respectively, for comparison with PBS (e) or indicated (g,h) by Bonferroni post-tests. Scale bars 1 cm (g) and 200 μM (h) Fig. 6 IKKα is required for mutantKRAS-induced malignant pleural effusion.a–cMalignant pleural disease induced by LLC cells (KrasG12C) stably expressing pNGLNF-κΒ reporter and control shRNA (shC) or shRNA targeting IKKα (shChuk), ΙΚΚβ (shIkbkb), ΙΚΚε (shIkbke), or TBK1 (shTbk1) transcripts (nis given in Table 3). Shown are Kaplan–Meier survival plot (a), data summaries of effusion volume and pleural fluid cells (b), and representative images of effusions (dashed lines) and pleural tumors (t) as well as bioluminescent images at day 13 after pleural injections of the indicated tumor cells (c).d–fMalignant pleural disease induced by MC38 cells (KrasG13R) stably expressing pNGLNF-κΒ reporter and shC, shChuk, or shIkbkb(nis given in Supplementary Table3). Shown are immunoblots of cytoplasmic extracts (d), data summaries of effusion volume and pleural fluid cells (e), and representative images of effusions (dashed lines) and pleural tumors (t) as well as representative bioluminescent images at day 13 after pleural injections of the indicated tumor cells (f).g–iMalignant pleural disease induced by PANO2 cells (KrasWT) stably expressing pNGLNF-κΒ reporter and control plasmid (shC) or plasmid encoding IKKα (pChuk), ΙΚΚβ (pIkbkb), or mutant (pKrasG12C) transcripts (nis given in Supplementary Table3). Shown are Kaplan–Meier survival plot (g), data summary of effusion volume (h), and representative images of effusions (dashed lines) and pleural tumors (t), hearts (h), and lungs (l), as well as representative bioluminescent images at day 14 after pleural injections of the indicated tumor cells (i). Data are presented as mean ± s.d.P, probability of no difference between cell lines by overall log-rank test (a,g) or one-way ANOVA (b,e,h). ns, single, double, and triple asterisks (*, **, and ***):P> 0.05,P< 0.05,P< 0.01, andP< 0.001, respectively, for the indicated comparisons with control cells by Bonferroni post-tests. Scale bars, 0.5 cm Kras G12C , Chuk , Ikbkb , Ikbke , and Tbk1 cDNAs were cloned via reverse transcriptase-PCR (RT-PCR) from LLC or MC38 RNA using specific primers (Supplementary Table 6 ) and were subcloned into peGFP-C1 (Takara, Mountain View, CA). eGFP , eGFP.Kras G12C , eGFP . 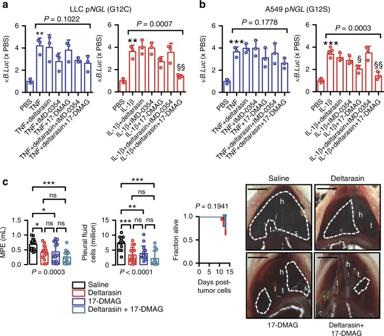Fig. 9 Combined targeting of mutantKRASand IKKα abolishes IL-1β-induced NF-κΒ activation and malignant pleural effusion development.a,bBioluminescent detection of NF-κΒ reporter activity in LLC (a;C57BL/6Lewis lung carcinoma,KrasG12C) and A549 (b; human lung adenocarcinoma,KrasG12S) cells stably expressing pNGLunder PBS or 1 nM TNF- or IL-1β-stimulated conditions (4 h), with or without pretreatment with 1 μM deltarasin, IMD-0354, or 17-DMAG alone or in combination (n= 3 independent experiments). Note four-fold induction of NF-κΒ reporter activity by both TNF and IL-1β. Note also inability of any treatment to block TNF-induced NF-κΒ activation and of any standalone treatment except 17-DMAG to inhibit IL-1β-induced NF-κΒ activation. Finally, note complete abrogation of IL-1β-induced NF-κΒ activation in both cell lines by deltarasin/17-DMAG combination. Data are presented as mean ± s.d.P, probability of no difference by one-way ANOVA (PBS group excluded). Double and triple asterisks (** and ***):P< 0.01 andP< 0.001, respectively, for comparison with PBS by Student’st-tests. Single and double section symbols (§ and §§):P< 0.05 andP< 0.01, respectively, for comparison with TNF or IL-1β by Bonferroni post-tests.cMalignant pleural disease induced by LLC cells in wild-typeC57BL/6mice treated with deltarasin and/or 17-DMAG. Mice received pleural LLC cells, were allowed 5 days for pleural tumor development, and were randomized to daily intraperitoneal treatments with saline (100 μL), deltarasin, 17-DMAG, or both (both at 15 mg/Kg in 100 μL saline;nis given in Supplementary Table3). Shown are data summaries of effusion volume and pleural fluid cells and Kaplan–Meier survival plot, as well as representative images of effusions (dashed lines), pleural tumors (t), lungs (l), and hearts (h). Data are presented as mean ± s.d.P, probability of no difference by one-way ANOVA or log-rank test. ns, single, double, and triple (*, **, and ***):P> 0.05,P< 0.05,P< 0.01, andP< 0.001, respectively, for the indicated comparisons by Bonferroni post-tests. Scale bars, 1 cm 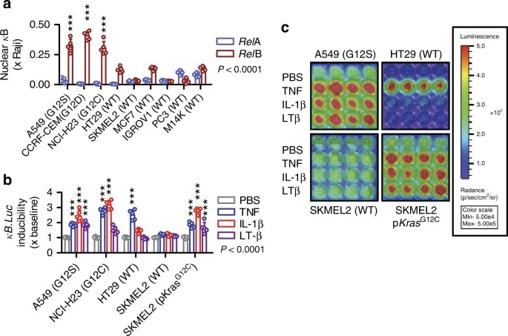Fig. 10 Non-canonical endogenous and IL-1β-inducible NF-κB activation ofKRAS-mutant human tumor cells. Different human cancer cell lines with (KRASMUT: A549,KRASG12S; CCRF-CEM,KRASG12D; NCI-H23,KRASG12C) or without (KRASWT; HT29, SKMEL2, MCF7, IGROV1, PC3, and M14K)KRASmutations were assessed for NF-κΒ activation at resting and stimulated conditions in vitro.aData summary (n= 5 independent experiments) of DNA NF-κB motif-binding activity of nuclear extracts by NF-κB ELISA relative to nuclear extracts of Raji leukemia cells. Note increased nuclearRelB and P52 binding activity ofKRASMUTcompared withKRASWTcells.b,cBioluminescent detection of NF-κΒ reporter activity in A549, NCI-H23, HT29, and SKMEL2 cells stably expressing pNGL, as well as in SKMEL2 cells stably expressing pNGLand pKrasG12C(b; data summary ofn= 5 independent experiments;c: representative bioluminescent images) during 4-h incubation with PBS or 1 nM TNF, IL-1β, or lymphotoxin (LT)-β. Note IL-1β-induced NF-κB activity ofKRASMUTbut not ofKRASWTcells. Note also instalment of IL-1β-induced NF-κB activation in SKMEL2 cells by pKrasG12C(SKMEL2 cells expressing pCbehaved exactly as parental cells). Data are presented as mean ± s.d.P, probability of no difference by two-way ANOVA. Triple astrisks (***):P< 0.001 for comparison withRelA (a) or PBS (b) by Bonferroni post-tests Chuk , eGFP . Ikbkb , eGFP . Ikbke , and eGFP . Tbk1 cDNAs were subcloned into the new retroviral expression vector (#58249, #64372,# 87033, #58251, #87444, and #87443, respectively). Retroviral particles were obtained by co-transfecting HEK293T cells with retroviral vectors, pMD2.G (#12259), and pCMV-Gag-Pol (Cell Biolabs, San Diego, CA) at 1.5:1:1 stoichiometry using CaCl 2 /BES. After 2 days, culture media were collected and applied to cancer cells. After 48 h, media were replaced by selection medium containing 2–10 μg/mL puromycin. Stable clones were selected and subcultured [11] . For stable plasmid/shRNA transfection, 10 5 tumor cells in six-well culture vessels were transfected with 5 μg DNA using Xfect (Takara), and clones were selected by G418 (400–800 μg/mL) or puromycin (2–10 μg/mL). Cellular assays In vitro cancer cell proliferation was determined using MTT assay. Nuclear extracts were assayed for Rel A, Rel B, c- Rel , P50, and P52 DNA-binding activity using a commercially available ELISA kit (Transam, Active Motif, Belgium). All cellular experiments were independently repeated at least thrice. Bioluminescence imaging Living cells and mice were imaged 0, 4, 8, 24, and 48 h after cellular treatments and 0 h, 4 h, and 12–14 days after pleural delivery of p NGL -expressing cells on a Xenogen Lumina II (Perkin-Elmer, Waltham, MA) after addition of 300 μg/mL D-luciferin to culture media or isoflurane anesthesia and delivery of 1 mg intravenous D-luciferin to the retro-orbital veins [8] , [9] , [10] , [11] , [16] , [25] , [34] , [35] . Data were analyzed using Living Image v.4.2 (Perkin-Elmer). qPCR and microarray RNA was isolated using Trizol (Invitrogen, Carlsbad, CA) and RNAeasy (Qiagen, Hilden, Germany) was reverse transcribed using Superscript III (Invitrogen), and RT-PCR or qPCR was performed using SYBR Green Master Mix in a StepOnePlus (Applied Biosystems, Carlsbad, CA) and specific primers (Supplementary Table 6 ). Ct values from triplicate qPCR reactions were analyzed by the 2 –ΔΔCT method [62] relative to Gusb mRNA levels. For microarray, RNA was extracted from triplicate cultures of 10 6 cells. Five micrograms pooled total RNA were quality tested on an ABI 2000 (Agilent Technologies, Sta. Clara, CA), labeled, and hybridized to GeneChip Mouse Gene 2.0 ST arrays (Affymetrix, St. Clara, CA). For analysis of differential gene expression ( Δ GE) and unsupervised hierarchical clustering, Affymetrix Expression and Transcriptome Analysis Consoles were used. Chromatin immunoprecipitation LLC cells were treated with PBS or 1 nM IL-1β, and 30 min later, cells were fixed sequentially with 2 mM di(N-succinimidyl) glutarate (Sigma) and 1% formaldehyde (Sigma) and quenched with 0.125 M glycine, followed by lysis with 1% sodium dodecyl sulfate (SDS), 10 mM EDTA, and 50 mM Tris pH 8. Sonication was performed in a Bioruptor (Diagenode) for 40 cycles (30 s on/off) power settings high), using 3 × 10 6 cells; 20 μg of chromatin was precipitated with 5 μg of Rel A, Rel B, IKKα, or IKKβ antibody or a mouse control immunoglobulin G (IgG). Immunoprecipitates were retrieved with 50 μl of magnetic Dynabeads conjugated to protein G (Invitrogen) and subjected to quantitative real-time PCR (Applied Biosystems StepOne), using the Kapa SYBR Fast qPCR Kit (KapaBiosystems, KK4605) for amplification of the Cxcl1 promoter or Gusb as control. The sequences of the primers used for Cxcl1 promoter are: 5′-ATACAGCAGGGTAGGGATGC, 3′-TTGCCAACTGTTTTTGTGG. The sequences of the primers used for Gusb are: 5′-TTACTTTAAGACGCTGATCACC, 3′-ACCTCCAAATGCCCATAGTC. BM cell derivation and transfer For adoptive BM replacement, Il1β−/− mice ( C57BL/6 background) received 10 million BM cells flushed from the femurs and tibias of C57BL/6 , Tnf−/− , or Il1β−/− donors ( C57BL/6 background) intravenously 12 h after total-body irradiation (1100 Rad) [11] , [25] , [34] , [35] . One mouse in each experiment was not engrafted (sentinel) and was observed till moribund between days 5 and 15 post-irradiation. The mice were left to be engrafted for 1 month, when full BM reconstitution is complete, before experimental induction of pleural carcinomatosis via intrapleural injection of LLC cells. 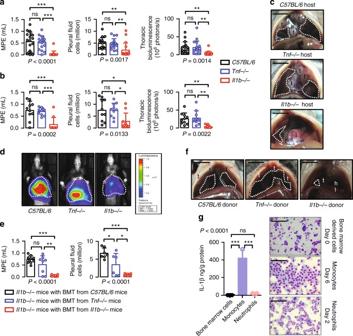For BM cell retrieval, BM cells were flushed from C57BL/6 femurs and tibias using full DMEM and were simply cultured in full culture media (the same used for cancer cell line cultures), supplemented with 20 ng/ml M-CSF or G-CSF in order for cells to differentiate to monocytes or neutrophils, respectively. Supernatants and cytocentrifugal specimens were obtained at day 0 for undifferentiated cells, day 2 for neutrophils, and at day 6 for monocytes/macrophages. Immunoblotting Nuclear and cytoplasmic extracts were prepared using the NE-PER Extraction Kit (Thermo, Waltham, MA), separated by 12% SDS polyacrylamide gel electrophoresis, and electroblotted to polyvinylidene difluoride membranes (Merck Millipore, Darmstadt, Germany). Fig. 7 Myeloid cell-derived IL-1β drives mutantKRAS-IKKα addiction in malignant pleural effusion.aMalignant pleural disease induced by LLC cells (KrasG12C) stably expressing pNGLNF-κΒ reporter plasmid in wild-typeC57BL/6mice (black) and TNF (blue) and IL-1β (red)-deficient mice (Tnf−/−andIl1b−/−, respectively; bothC57BL/6background;nis given in Supplementary Table3). Shown are data summaries of effusion volume, pleural fluid cells, and NF-κΒ-dependent thoracic bioluminescent signal.b–dMalignant pleural disease induced by MC38 cells (KrasG13R) stably expressing pNGLNF-κΒ reporter plasmid in wild-typeC57BL/6(black),Tnf−/−(blue), andIl1b−/−(red) mice (allC57BL/6background;nis given in Supplementary Table3). Shown are data summaries of effusion volume, pleural fluid cells, and NF-κΒ-dependent thoracic bioluminescent signal (b), representative images of effusions (dashed lines), pleural tumors (t), and lungs (l) (c), as well as representative bioluminescent images at day 13 after pleural injections of the indicated tumor cells (d).e,fMalignant pleural disease induced by LLC cells inIl1b−/−mice (C57BL/6background;nis given in Supplementary Table3) that received total body irradiation (1100 Rad), same-day bone marrow transplants (10 million cells) fromC57BL/6(black),Tnf−/−(blue), orIl1b−/−(red) donors, and pleural tumor cells after 1 month. Shown are data summaries of effusion volume and pleural fluid cells (e) and representative images of effusions (dashed lines), pleural tumors (t), lungs (l), and hearts (h) (f).gIL-1β protein secretion byC57BL/6mouse bone marrow-isolated myeloid cells 24 h after treatment with LLC supernatants; undifferentiated cells (day 0), neutrophils (day 2 after addition of 20 ng/ml G-CSF), and macrophages (day 6 after addition of 20 ng/ml M-CSF;n= 3 independent experiments). Data are presented as mean ± s.d.P, probability of no difference by one-way ANOVA. ns, single, double, and triple asterisks (*, **, and ***):P> 0.05,P< 0.05,P< 0.01, andP< 0.001, respectively, for the indicated comparisons by Bonferroni post-tests. Scale bars, 1 cm (c,f) and 100 μM (g) Membranes were probed with specific antibodies (Supplementary Table 7 ) and were visualized by film exposure after incubation with enhanced chemiluminescence substrate (Merck Millipore, Darmstadt, Germany). Electrophoretic mobility shift assay (EMSA) Nuclear extracts were prepared using the NE-PER Extraction Kit. Proteins (10 μg) were incubated with NF-κB biotin-labeled probe using a commercially available non-radioactive EMSA Kit (Signosis Inc, Santa Clara, USA). DNA–protein complexes were electrophoresed in a prerinsed 6.5% polyacrylamide gel, transferred to a positively charged nylon membrane, and were visualized by film exposure after incubation with enhanced chemiluminescence substrate. For gel shift reactions, proteins were incubated with the specific antibody for 1 h at 4 °C before probe incubation. The antibodies used for observing the supershifted bands were Rel A and Rel B. IgG antibody served as negative control for super-shift assays. Immunofluorescence For immunofluorescence, cells were fixed in 4% paraformaldehyde overnight at 4 °C and were labeled with the indicated primary antibodies (Supplementary Table 7 ) followed by incubation with fluorescent secondary antibodies (Invitrogen, Waltham, MA; Supplementary Table 7 ). Cells were then counterstained with Hoechst 33258 (Sigma-Aldrich, St. Louis, MO) and mounted with Mowiol 4-88 (Calbiochem, Gibbstown, NJ). For isotype control, the primary antibody was omitted. Fluorescent microscopy was carried out on an AxioObserver.D1 inverted microscope (Zeiss, Jena, Germany) connected to an AxioCam ERc 5 s camera (Zeiss), and digital images were processed with the Fiji academic imaging freeware [63] . Statistics Sample size was calculated using G*power ( http://www.gpower.hhu.de/ ) [64] assuming α = 0.05, β = 0.05, and d = 1.5, tailored to detect 30% differences between means with 20–30% SD spans, yielding n = 13/group. Animals were allocated to groups by alternation (treatments or cells) or case–control-wise (transgenic animals). Data acquisition was blinded on samples coded by non-blinded investigators. No data were excluded. All data were examined for normality by Kolmogorov–Smirnof test and were normally distributed. Values are given as mean ± SD. Sample size ( n ) refers to biological replicates. Differences in means were examined by t -test and one-way or two-way ANOVA with Bonferroni post-tests, in frequencies by Fischer’s exact or χ 2 tests, and in Kaplan–Meier survival estimates by log-rank test, as appropriate. P -values are two-tailed. P < 0.05 was considered significant. Analyses and plots were done on Prism v5.0 (GraphPad, La Jolla, CA). Data availability All new plasmids have been deposited at the Addgene plasmid repository ( https://www.addgene.org/search/advanced/?q=stathopoulos ) and their IDs (#) are given in the text. Microarray data are available at the GEO ( http://www.ncbi.nlm.nih.gov/geo/ ; Accession IDs: GSE93369 and GSE93370). The authors declare that all the other data supporting the findings of this study are available within the article and its supplementary information files and from the corresponding authors upon reasonable request.